Facultative CTCF sites moderate mammary super-enhancer activity and regulate juxtaposed gene in non-mammary cells Precise spatiotemporal gene regulation is paramount for the establishment and maintenance of cell-specific programmes. Although there is evidence that chromatin neighbourhoods, formed by the zinc-finger protein CTCF, can sequester enhancers and their target genes, there is limited in vivo evidence for CTCF demarcating super-enhancers and preventing cross talk between distinct regulatory elements. Here, we address these questions in the Wap locus with its mammary-specific super-enhancer separated by CTCF sites from widely expressed genes. Mutational analysis demonstrates that the Wap super-enhancer controls Ramp3 , despite three separating CTCF sites. Their deletion in mice results in elevated expression of Ramp3 in mammary tissue through augmented promoter–enhancer interactions. Deletion of the distal CTCF-binding site results in loss of Ramp3 expression in non-mammary tissues. This suggests that CTCF sites are porous borders, allowing a super-enhancer to activate a secondary target. Likewise, CTCF sites shield a widely expressed gene from suppressive influences of a silent locus. Super-enhancers control lineage-specific genes [1] , [2] , [3] , [4] , [5] and activate them up to several thousand-fold [6] . In order to prevent a spill over of transcriptional activity, such loci need to be self-contained units and demarcated from neighbouring genes that are subject to their own distinct control. This ensures that neighbouring non-target genes are correctly regulated. Equally important, active genetic units need to be impervious to flanking heterochromatin to avoid inappropriately silencing. Experimental evidence suggests that genes and their associated regulatory elements are located within genetically confined neighbourhoods [7] , [8] , [9] , [10] , [11] , [12] . The concept of a genome compartmentalized into regulatory neighbourhoods [7] , [8] , [9] , [10] , [11] , [12] , such as topological-associated domains (TADs) [9] , [11] and insulated neighbourhoods [7] , [8] , [12] , was established along with the identification of chromatin loops using Chromosome Conformation Capture (3C) technologies, Chromatin Interaction Analysis by Paired-End Tag sequencing (ChIA-PET) [13] and Hi-C [14] , and the accompanying computational approaches. Such regulatory neighbourhoods not only limit the search space of cis -regulatory elements to genes within the same domain but also prevent active and suppressive chromatin from spreading [7] , [15] , [16] , [17] , [18] . The zinc-finger protein CTCF, which is known for its insulator function [19] , [20] , [21] , has been shown to be instrumental in establishing such insulated neighbourhoods [7] and is also enriched at TAD borders [9] . High-resolution data suggest a size of approximately 185 kb for TADs [22] , called contact domains [22] . The additional presence of sub-domain chromatin loops within TADs enables accurate promoter–enhancer interactions necessary for the developmental control of resident genes [22] . Current knowledge about biological functions of CTCF sites has been obtained mainly from studies on cell lines and embryonic stem cells (ESCs) [7] , [10] , [15] , [16] , [18] , [23] , [24] , [25] , [26] . Only a limited number of mouse studies have been conducted [17] , [25] , [27] , [28] , [29] , [30] , [31] and these have in general not addressed the extent to which CTCF sites can shield non-target genes from juxtaposed enhancers. Naturally occurring human mutations and engineered mice carrying the mutations in CTCF sites have provided additional information on their contribution in developmental diseases and tumorigenesis [17] , [26] , [31] , [32] , [33] , [34] , [35] , [36] . However, there has been no genetic assessment of the contribution of CTCF sites in confining cell-specific and cytokine-sensing enhancers in a genuine in vivo setting. Cytokine-sensing super-enhancers can activate genes up to several thousand-fold and it is not clear whether CTCF sites can demarcate them to avoid aberrant regulation of outside genes. In a quest to understand the physiological role of CTCF in the cell-specific control of super-enhancers, we turned to the mammary gland, whose sole purpose is the production of milk to nourish the young. More than 90% of the protein content of milk is contributed by less than 10 proteins [37] and expression of the respective genes in alveolar epithelium is induced up to 1,000-fold during pregnancy [38] . The extraordinary expression levels of milk protein genes are the result of mammary-specific super-enhancers that integrate prolactin signalling during pregnancy and lactation [6] . While highly active in mammary alveolar epithelium, most milk protein encoding genes are virtually silent in non-mammary cells, even in those that sense cytokines including prolactin. Mammary-specific genes are surrounded by genes expressed across cell types and are subject to their own regulatory features. It is essential that mammary super-enhancers only activate their respective target genes and neighbouring off-target genes remain inert to their influence. Inadvertent and exorbitant expression of any biologically active protein in mammary tissue could be detrimental to its physiology [39] . Since mammary enhancers are composed of common elements that can be activated by many cytokines, it is essential to shield their influence from neighbouring genes in non-mammary cells. Equally important, it is vital that the transcriptional silence of mammary loci in non-mammary cells does not spread to active neighbouring genes, which could result in their inadvertent silencing with all its potential consequences. At this point it is not known whether CTCF sites demarcate highly active mammary super-enhancers from neighbouring genes. Here, we have used the well-characterized Wap locus to investigate the biological role of CTCF sites controlling mammary-specific loci. The Wap gene itself is expressed exclusively in mammary epithelium and its more than 1,000-fold activation during pregnancy is controlled by a tripartite super-enhancer that senses prolactin through the transcription factor STAT5 and likely other mammary-enriched transcription factors [6] . The Wap locus is compact and Ramp3 , which is expressed in many cell types at low levels, is located within 14 kb of the super-enhancer. Tbrg4 , which is also expressed at low levels in many cell types, flanks the other side of the Wap locus. Both RAMP3 (ref. 40 ) and TBRG4 [41] are regulatory proteins and well-defined levels likely ensure biological functions of expressing cells. We identify five CTCF-binding sites in mammary tissue that separate the Wap gene with its super-enhancer from its neighbouring genes using ChIP-seq. Based on these findings we address four specific questions. Is the Wap gene located within a unique regulatory domain separated from neighbouring genes? Does the Wap super-enhancer activate the two neighbouring non-target genes in mammary tissue? Do CTCF sites shield the Wap super-enhancer from neighbouring genes in mammary tissue? Do CTCF sites shield the silent Wap gene in non-mammary cells from common regulatory elements controlling the two neighbouring genes? We demonstrate that CTCF sites do not constitute a tight genetic boundary encapsulating the mammary-specific Wap super-enhancer and its associated gene, but are a porous border that tolerates enhancer spill over to the neighbouring non-target Ramp3 gene. We also demonstrate that a conserved CTCF site separating the Wap super-enhancer from the Ramp3 gene is required for Ramp3 expression in non-mammary tissues. We show that CTCF-binding sites contribute to cell-specific functions in the activation and silencing of genes. Identification of CTCF sites associated with super-enhancers Mammary super enhancers activate their respective target genes up to 1,000-fold during pregnancy but have little or no impact on neighbouring non-target genes [6] . To investigate the possibility that the zinc-finger protein CTCF contributes to shielding mammary enhancers from non-target genes, we initially analysed genome-wide binding of CTCF in mammary tissue at day one of lactation ( Fig. 1 ). ChIP-seq experiments demonstrated the presence of approximately 26,200 CTCF-binding sites. Based on a comparison with published ChIP-seq data from other tissues, 98% of these binding sites were shared with those found in one or more tissues (Th17 cells, kidney, heart, cerebellum and adipose tissue) and 2% (588) appeared to be mammary-specific. CTCF-binding sites shared between tissues were distinct from mammary-specific sites ( Fig. 1b ). Shared sites had on average a 1.6-fold higher read coverage than mammary-specific sites ( Fig. 1b ). While 74% of the common peaks displayed a bona fide binding motif, so did 57% of the mammary-specific ones ( Fig. 1c ). 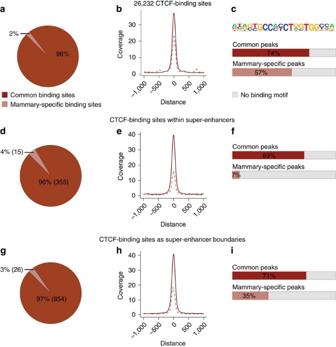Figure 1: Global analysis of CTCF-binding sites. A total of 26,232 CTCF-binding sites were identified by ChIP-seq of mammary tissue from lactating mice, by peak calling and overlapping three CTCF ChIP-seq samples (a) Ninety-eight per cent (25,644) of the sites were shared between mammary tissue, adipose tissue, cerebellum, heart, kidney and Th17 cells (GSE29218, GSE40918, GSE74189, GSE74826). Out of those, 65% (16,733) have been identified in all tissues and 35% (8,911) in distinct subsets. Two per cent (588) of the sites appeared to be mammary-specific. (b) Read coverage of CTCF-binding sites shared between tissues (height 37) was approximately 1.6 times higher than the mammary-specific ones (height 23). (c) The CCCTC motif was the highest ranked motif in both peak sets (±200 bp). Seventy-four per cent (19,057) of CTCF-binding sites shared between tissues had an underlying CCCTC-binding motif and 57% (337) of the mammary-specific binding sites had one. (d) A total of 370 CTCF-binding sites were detected within the 440 mammary super-enhancers. Ninety-six per cent (355) of them were shared CTCF-binding sites and 4% (15) were mammary-specific. (e) The read coverage of CTCF-binding sites shared between tissues (height 40) was approximately 2.5 times higher than those of mammary-specific ones (height 16). (f) Sixty-nine per cent (246) of the shared CTCF-binding sites and one site (7%) of the mammary-specific ones had an underlying CTCF motif. (g) CTCF-binding sites associated with 440 mammary super-enhancer boundaries. Ninety-seven per cent (854) were shared between tissues and 3% (26) were mammary-specific. (h) Read coverage of CTCF-binding sites shared between tissues (height 41) was approximately two times higher than that of mammary-specific ones (height 19). (i) Seventy-one per cent (610) of shared CTCF-binding sites, and 35% (nine) of mammary-specific ones had an underlying CTCF motif. Figure 1: Global analysis of CTCF-binding sites. A total of 26,232 CTCF-binding sites were identified by ChIP-seq of mammary tissue from lactating mice, by peak calling and overlapping three CTCF ChIP-seq samples ( a ) Ninety-eight per cent (25,644) of the sites were shared between mammary tissue, adipose tissue, cerebellum, heart, kidney and Th17 cells (GSE29218, GSE40918, GSE74189, GSE74826). Out of those, 65% (16,733) have been identified in all tissues and 35% (8,911) in distinct subsets. Two per cent (588) of the sites appeared to be mammary-specific. ( b ) Read coverage of CTCF-binding sites shared between tissues (height 37) was approximately 1.6 times higher than the mammary-specific ones (height 23). ( c ) The CCCTC motif was the highest ranked motif in both peak sets (±200 bp). Seventy-four per cent (19,057) of CTCF-binding sites shared between tissues had an underlying CCCTC-binding motif and 57% (337) of the mammary-specific binding sites had one. ( d ) A total of 370 CTCF-binding sites were detected within the 440 mammary super-enhancers. Ninety-six per cent (355) of them were shared CTCF-binding sites and 4% (15) were mammary-specific. ( e ) The read coverage of CTCF-binding sites shared between tissues (height 40) was approximately 2.5 times higher than those of mammary-specific ones (height 16). ( f ) Sixty-nine per cent (246) of the shared CTCF-binding sites and one site (7%) of the mammary-specific ones had an underlying CTCF motif. ( g ) CTCF-binding sites associated with 440 mammary super-enhancer boundaries. Ninety-seven per cent (854) were shared between tissues and 3% (26) were mammary-specific. ( h ) Read coverage of CTCF-binding sites shared between tissues (height 41) was approximately two times higher than that of mammary-specific ones (height 19). ( i ) Seventy-one per cent (610) of shared CTCF-binding sites, and 35% (nine) of mammary-specific ones had an underlying CTCF motif. Full size image Next, we investigated the possibility that mammary super-enhancers were associated with specific CTCF sites. Ninety-six per cent of the 370 CTCF sites located within the 440 mammary super-enhancers [6] were shared with several cell types (Fig. 1d) and their read coverage exceeded that of mammary-specific sites by 2.5-fold ( Fig. 1e ). Moreover, while 69% of the shared sites had a CTCF recognition motif, only 7% of the mammary-specific ones displayed one ( Fig. 1f ). Similarly, 97% of the 854 CTCF sites flanking mammary super-enhancers were shared with other tissues ( Fig. 1g ), their peak coverage was higher than that of mammary-specific ones ( Fig. 1h ) and 71% of those shared binding sites had a CTCF motif ( Fig. 1i ). In summary, most CTCF-binding sites associated with mammary super-enhancers are not unique to mammary tissue. The Wap super-enhancer activates the juxtaposed Ramp3 gene We have recently identified and dissected a complex mammary super-enhancer that activates the Wap gene more than 1,000-fold during pregnancy [6] . The extended locus contains the Wap gene, whose expression is confined to mammary epithelium, and two genes, Ramp3 and Tbrg4 , which are active across cell types. This locus contains at least five CTCF sites that are shared between different cell types ( Fig. 2a ). CTCF binding to site A, which coincides with a TAD boundary [9] , and sites E and F, which presumably serve as loop anchors [7] , [22] , were conserved across cell types ( Fig. 2a,b ). CTCF binding to sites C and D was preferentially found in cells that respond to cytokines, such as T cells. 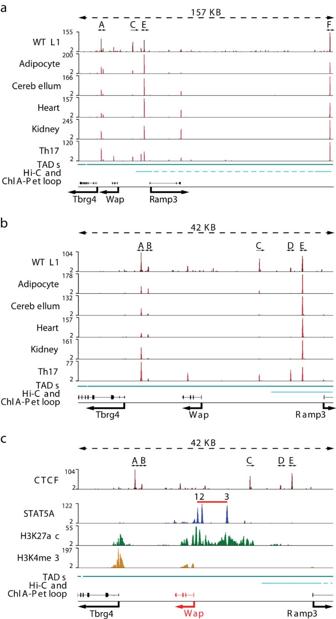Figure 2: CTCF-binding sites and enhancers in the extendedWaplocus. (a) CTCF ChIP-seq data from mammary tissue at day 1 of lactation and from several non-mammary cells (GSE29218, GSE40918, GSE74189, GSE74826). The lower part shows the topological associated domain9(TAD) (bin size 40KB) in cyan and a ChIA-PET and Hi-C loop7with site E and F as anchor in light blue. (b) CTCF binding to sites A and F was conserved across cell types. CTCF binding to sites B, C and D was cell-preferential. (c) TheWaplocus is characterized by its tripartite mammary-specific super-enhancer (shown as red bar) and five flanking CTCF sites (GSE74826), which separate it from the two neighbouring genes,Tbrg4andRamp3. Both are expressed at low levels (FPKM<13) in mammary tissue.Ramp3is preferentially expressed in the cerebellum, whereasTbrg4is widely expressed. Two CTCF-binding sites are 3′ of theWapgene body and three 5′ sites are located between the super-enhancer andRamp3. TheWaplocus is located within a topological-associated domain9(TAD) (bin size 40KB). CTCF site E anchors a ChIA-PET and Hi-C loop7. Figure 2: CTCF-binding sites and enhancers in the extended Wap locus. ( a ) CTCF ChIP-seq data from mammary tissue at day 1 of lactation and from several non-mammary cells (GSE29218, GSE40918, GSE74189, GSE74826). The lower part shows the topological associated domain [9] (TAD) (bin size 40KB) in cyan and a ChIA-PET and Hi-C loop [7] with site E and F as anchor in light blue. ( b ) CTCF binding to sites A and F was conserved across cell types. CTCF binding to sites B, C and D was cell-preferential. ( c ) The Wap locus is characterized by its tripartite mammary-specific super-enhancer (shown as red bar) and five flanking CTCF sites (GSE74826), which separate it from the two neighbouring genes, Tbrg4 and Ramp3 . Both are expressed at low levels (FPKM<13) in mammary tissue. Ramp3 is preferentially expressed in the cerebellum, whereas Tbrg4 is widely expressed. Two CTCF-binding sites are 3′ of the Wap gene body and three 5′ sites are located between the super-enhancer and Ramp3 . The Wap locus is located within a topological-associated domain [9] (TAD) (bin size 40KB). CTCF site E anchors a ChIA-PET and Hi-C loop [7] . Full size image Based on Hi-C [22] and ChIA-PET [7] data sets, Ramp3 is located within its own distinct chromatin loop separated from the highly active Wap gene ( Fig. 2c ). Notably, H3K27ac marks covering the Wap super-enhancer did not extend past bordering CTCF sites into the Ramp3 locus ( Fig. 2c ). However, these structural data provided no information on the extent to which Wap super-enhancer elements could activate the neighbouring Ramp3 gene. RNA-seq experiments [38] demonstrated that while Wap was induced 1,000-fold between day 6 of pregnancy and day 1 of lactation, Ramp3 mRNA levels increased approximately five-fold ( Fig. 3a ). In contrast, Tbrg4 mRNA levels remained constant. This suggests the possibility that Ramp3 is controlled to some extent by the juxtaposed Wap super-enhancer. Alternatively, the increase of Ramp3 mRNA levels during pregnancy could merely reflect an increased proportion of secreting epithelial cells, which might preferentially express Ramp3 . 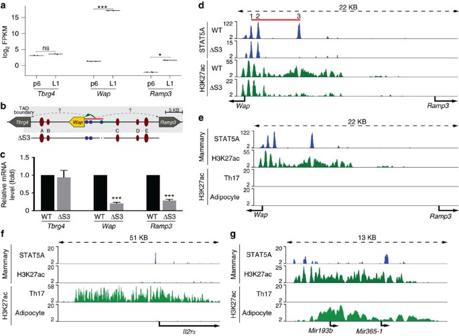Figure 3:Wapsuper-enhancer activates theRamp3gene. (a) RNA-seq data from mammary tissue at day 6 of pregnancy (p6) and day 1 of lactation (L1) demonstrated thatWapandRamp3are induced during pregnancy, althoughRamp3is expressed at a much lower level.Tbrg4expression remained unchanged (GSE37646). Results are shown as box plots; median, middle bar inside the box; IQR, 50% of the data; whiskers, 1.5 times the IQR; p6:n=3 and L1:n=2. Student’st-test with alpha 0.01 was applied for p6 and L1 for each gene independently. *P<0.01, **P<0.001, ***P<0.0001. (b) The cartoon illustratesWapand its flanking genes. The blue circles represent the constituent enhancers of the super-enhancer (shown as red bar). H3K27ac is shown in green. The crimson ovals represent the sites bound by CTCF. (c) Gene expression data from the enhancer mutant ΔS3 demonstrated thatRamp3expression was reduced by 70%. Results are shown as the means±s.e.m. of independent biological replicates; ΔS3:n=3; data were normalized toGapdh; a two-tailed Student’st-test was applied with alpha 0.01 for wild type and ΔS3 for each gene independently. *P<0.01, **P<0.001, ***P<0.0001. (d) STAT5 binding and H3K27ac in theWap-Ramp3locus in WT and ΔS3 mutant mammary tissue (GSE74826). (e) H3K27ac at theWap-Ramp3locus in mammary tissue, Th17 cells and adipocytes (GSE90788, GSE92590). (f) H3K27ac at theIl2rαlocus in mammary tissue, Th17 cells and adipocytes. (g) H3K27ac at theMir193blocus in mammary tissue, Th17 cells and adipocytes. Figure 3: Wap super-enhancer activates the Ramp3 gene. ( a ) RNA-seq data from mammary tissue at day 6 of pregnancy (p6) and day 1 of lactation (L1) demonstrated that Wap and Ramp3 are induced during pregnancy, although Ramp3 is expressed at a much lower level. Tbrg4 expression remained unchanged (GSE37646). Results are shown as box plots; median, middle bar inside the box; IQR, 50% of the data; whiskers, 1.5 times the IQR; p6: n =3 and L1: n =2. Student’s t -test with alpha 0.01 was applied for p6 and L1 for each gene independently. * P <0.01, ** P <0.001, *** P <0.0001. ( b ) The cartoon illustrates Wap and its flanking genes. The blue circles represent the constituent enhancers of the super-enhancer (shown as red bar). H3K27ac is shown in green. The crimson ovals represent the sites bound by CTCF. ( c ) Gene expression data from the enhancer mutant ΔS3 demonstrated that Ramp3 expression was reduced by 70%. Results are shown as the means±s.e.m. of independent biological replicates; ΔS3: n =3; data were normalized to Gapdh ; a two-tailed Student’s t -test was applied with alpha 0.01 for wild type and ΔS3 for each gene independently. * P <0.01, ** P <0.001, *** P <0.0001. ( d ) STAT5 binding and H3K27ac in the Wap-Ramp3 locus in WT and ΔS3 mutant mammary tissue (GSE74826). ( e ) H3K27ac at the Wap-Ramp3 locus in mammary tissue, Th17 cells and adipocytes (GSE90788, GSE92590). ( f ) H3K27ac at the Il2rα locus in mammary tissue, Th17 cells and adipocytes. ( g ) H3K27ac at the Mir193b locus in mammary tissue, Th17 cells and adipocytes. Full size image We investigated the possibility that Ramp3 is under control of the juxtaposed Wap super-enhancer, which is composed of three constituent enhancers ( Fig. 3b ), with the most distal S3 accounting for 90% of its activity [6] . Deletion of S3 (ΔS3) resulted in an approximately 70% reduction of Ramp3 mRNA in mammary tissue ( Fig. 3c ). Although Wap and Ramp3 are expressed at vastly different levels in mammary tissue, the relative impact of the super-enhancer was equivalent on both genes despite the presence of three CTCF sites separating it from Ramp3 . Since wild type and mutant mammary tissues were obtained from lactating mice, we can exclude the possibility that non-mammary cells were responsible for the differential Ramp3 expression between pregnancy and lactation. While the Wap super-enhancer and its associated regulatory regions are characterized by extensive H3K27ac, few, if any, of these marks were detected over the Ramp3 gene ( Fig. 3d ). H3K27ac coverage of the Wap region was greatly reduced in ΔS3 mammary tissue and absent at the Ramp3 gene [6] ( Fig. 3d ). The Ramp3 gene also displayed a paucity of H3K27ac marks in Th17 cells and adipose tissue ( Fig. 3e ) reflecting low expression levels. The Il2rα gene served as a positive H3K27ac control in Th17 cells ( Fig. 3f ) and Mir193b (ref. 42 ) in adipocytes ( Fig. 3g ). Tbrg4 mRNA levels were not significantly reduced in ΔS3 mutant mammary tissue, suggesting spatial selectivity of the S3 enhancer. Of note, the vastly higher expression of Wap compared to Ramp3 might be caused by additional regulatory elements or differential stability of the two mRNAs. CTCF sites moderate super-enhancer activity Although the S3 enhancer of the Wap super-enhancer activates Ramp3 despite the presence of three separating CTCF sites, it is not clear to what extent these sites muffle super-enhancer activity. To investigate this, we deleted these CTCF sites individually and in combination from the mouse genome ( Fig. 4 ). While CTCF binding to site E, an anchor of the loop that encapsulates Ramp3 , is conserved across all cell types analysed ( Fig. 2a ), CTCF binding to sites C and D is also found in a subset of cells, such as T cells. In addition to these three sites we also investigated the two CTCF-binding sites demarcating the Wap gene from its downstream neighbour Tbrg4 ( Fig. 4a ). Deletion of these two sites in the mouse germline resulted in the loss of CTCF binding ( Fig. 4b ) but did not result in an altered expression of Tbrg4 or Wap in lactating mammary tissue ( Fig. 4c ). This suggests that the Wap super-enhancer is unable to regulate Tbrg4 , which is in accordance with studies in other systems [25] . Alternatively, a weak CTCF-binding site located in the third intron of the Wap gene could function as a boundary element. 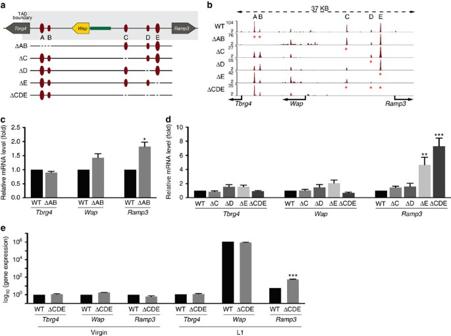Figure 4: Deletion of CTCF sites flanking theWaplocus. (a) Diagram of the CTCF-binding sites in theTbrg4-Wap-Ramp3locus and the deletions investigated. Individual deletions of sites C, D and E and two combined deletions, one comprising sites A and B and one comprising sites C, D and E were generated and analysed. (b) CTCF ChIP-seq analyses from mutant tissues confirmed loss of CTCF binding at the respective deleted sites. (c) Deletion of sites A and B did not affect expression ofTbrg4andWapusing qRT–PCR. Results are shown as the means±s.e.m. of independent biological replicates; ΔABn=4 (−/−); data were normalized toGapdh; a two-tailed Student’st-test was applied with alpha 0.01 for wild type and ΔAB for each gene independently. *P<0.01, **P<0.001, ***P<0.0001. (d)Tbrg4,WapandRamp3mRNA levels in lactating mammary tissue lacking CTCF sites separating these two genes. Loss of sites C or D did not affect gene expression, whereas loss of site E resulted in an approximately five-fold increase in expression ofRamp3and a seven-fold induction in mice carrying combined deletions of C, D and E.Tbrg4andWapdid not show changes in gene expression. Results are shown as the means±s.e.m. of independent biological replicates; ΔCn=10 (−/−); ΔDn=5 (−/−); ΔEn=7 (−/−); ΔCDE:n=4 (−/−); data were normalized toGapdh; one-way ANOVA with multiple comparison and alpha 0.01 was applied. *P<0.01, **P<0.001, ***P<0.0001; (e)Tbrg4,WapandRamp3mRNA levels in virgin mammary tissue lacking the three CTCF sites separating theWapsuper-enhancer from theRamp3gene. A two-tailed Student’st-test was applied with alpha 0.01 for wild type and ΔCDE for each gene independently. *P<0.01, **P<0.001, ***P<0.0001. Figure 4: Deletion of CTCF sites flanking the Wap locus. ( a ) Diagram of the CTCF-binding sites in the Tbrg4-Wap-Ramp3 locus and the deletions investigated. Individual deletions of sites C, D and E and two combined deletions, one comprising sites A and B and one comprising sites C, D and E were generated and analysed. ( b ) CTCF ChIP-seq analyses from mutant tissues confirmed loss of CTCF binding at the respective deleted sites. ( c ) Deletion of sites A and B did not affect expression of Tbrg4 and Wap using qRT–PCR. Results are shown as the means±s.e.m. of independent biological replicates; ΔAB n =4 (−/−); data were normalized to Gapdh ; a two-tailed Student’s t -test was applied with alpha 0.01 for wild type and ΔAB for each gene independently. * P <0.01, ** P <0.001, *** P <0.0001. ( d ) Tbrg4 , Wap and Ramp3 mRNA levels in lactating mammary tissue lacking CTCF sites separating these two genes. Loss of sites C or D did not affect gene expression, whereas loss of site E resulted in an approximately five-fold increase in expression of Ramp3 and a seven-fold induction in mice carrying combined deletions of C, D and E. Tbrg4 and Wap did not show changes in gene expression. Results are shown as the means±s.e.m. of independent biological replicates; ΔC n =10 (−/−); ΔD n =5 (−/−); ΔE n =7 (−/−); ΔCDE: n =4 (−/−); data were normalized to Gapdh ; one-way ANOVA with multiple comparison and alpha 0.01 was applied. * P <0.01, ** P <0.001, *** P <0.0001; ( e ) Tbrg4 , Wap and Ramp3 mRNA levels in virgin mammary tissue lacking the three CTCF sites separating the Wap super-enhancer from the Ramp3 gene. A two-tailed Student’s t -test was applied with alpha 0.01 for wild type and ΔCDE for each gene independently. * P <0.01, ** P <0.001, *** P <0.0001. Full size image We asked whether the three CTCF sites separating the Wap super-enhancer from Ramp3 have any inherent insulating capacity and deleted them in mice using CRISPR/Cas9 gene editing ( Fig. 4a ). Loss of CTCF binding in the different mutants was confirmed by ChIP-seq experiments ( Fig. 4b ). Next, we investigated the impact of individual deletions on the expression of Wap and Ramp3 in mammary tissue ( Fig. 4d ). None of the individual or combined deletions impacted Wap expression at the onset of lactation ( Fig. 4d ). However, a differential impact on the neighbouring Ramp3 gene was obtained ( Fig. 4d ). While loss of sites C or D was inconsequential for Ramp3 expression, loss of site E resulted in an approximately five-fold induction of Ramp3 ( Fig. 4d ). Even though site E seems to be the only one to individually muffle Wap super-enhancer activity, we also investigated the consequences upon loss of all three sites. The combined loss of these sites resulted in an approximately seven-fold increase of Ramp3 mRNA ( Fig. 4d ). This suggests that sites C and D have measurable biological activity only in the context of site E. Although milk-secreting cells constitute the vast majority of mammary epithelium during lactation, it is possible that Ramp3 is expressed at significant levels in other cell types. To account for this, we analysed Wap and Ramp3 mRNA levels in mammary tissue from non-parous mice ( Fig. 4e ). The combined loss of CTCF sites C, D and E did not significantly alter the expression of Wap and Ramp3 genes in mammary tissue from virgin mice, suggesting that the transcriptional activation of the Ramp3 gene during pregnancy is the result of Wap enhancer activity. We further examined the possibility that this induction was the result of an expansion of Wap super-enhancer structures. Notably, the combined loss of sites C, D and E resulted in elevated H3K27ac over the Ramp3 gene ( Fig. 5a ). De novo H3K27ac acquisition was preferentially obtained in the first intron of Ramp3 and coincided with increased CTCF binding in these mutants ( Fig. 6b ). We also observed an expansion of H3K27ac in mammary tissue lacking only site C, which directly borders the Wap super-enhancer. However, this enhanced H3K27ac, which extended to site E, was without measurable consequences on gene expression ( Fig. 4d ). The H3K27ac pattern at the Bcl6 locus served as control accommodating variations between samples ( Fig. 5b ). Densitometry of H3K27ac occupancy supported the expansion of enhancer marks into the Ramp3 locus ( Fig. 5c,d ). 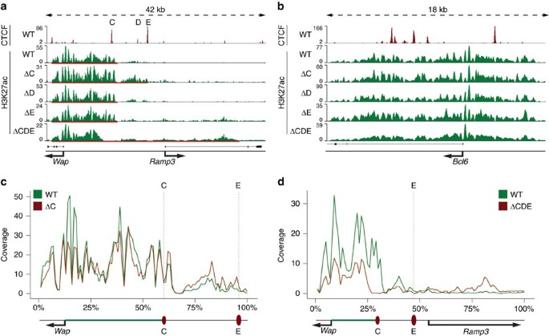Figure 5: Expansion of H3K27ac marks upon deletion of CTCF sites. ChIP-seq was used to identify changes of H3K27ac due to mutated CTCF-binding sites. (a) Deletion of CTCF site C resulted in the expansion of H3K27ac associated with theWapsuper-enhancer (red bar). This was not observed upon loss of sites D or E. The combined loss of sites C, D and E resulted also in an expansion of H3K27ac and was particular strong at a specific site in the first intron ofRamp3(normalized to 10 million reads) (red bar). (b) H3K27ac intensity was equivalent in the unrelatedBcl6locus. (c) H3K27ac profiles of theWap-Ramp3locus based on the data shown ina. Green, WT pattern; red, ΔC. The degree of H3K27ac in mutants was elevated between CTCF sites C and E confirming the expansion of H3K27ac (normalized to 10 million reads). (d) H3K27ac profiles of the data shown ina. WT is shown in green, ΔCDE in red. H3K27ac marks spread from site E to the second exon ofRamp3(normalized to 10 million reads). Figure 5: Expansion of H3K27ac marks upon deletion of CTCF sites. ChIP-seq was used to identify changes of H3K27ac due to mutated CTCF-binding sites. ( a ) Deletion of CTCF site C resulted in the expansion of H3K27ac associated with the Wap super-enhancer (red bar). This was not observed upon loss of sites D or E. The combined loss of sites C, D and E resulted also in an expansion of H3K27ac and was particular strong at a specific site in the first intron of Ramp3 (normalized to 10 million reads) (red bar). ( b ) H3K27ac intensity was equivalent in the unrelated Bcl6 locus. ( c ) H3K27ac profiles of the Wap-Ramp3 locus based on the data shown in a . Green, WT pattern; red, ΔC. The degree of H3K27ac in mutants was elevated between CTCF sites C and E confirming the expansion of H3K27ac (normalized to 10 million reads). ( d ) H3K27ac profiles of the data shown in a . WT is shown in green, ΔCDE in red. H3K27ac marks spread from site E to the second exon of Ramp3 (normalized to 10 million reads). 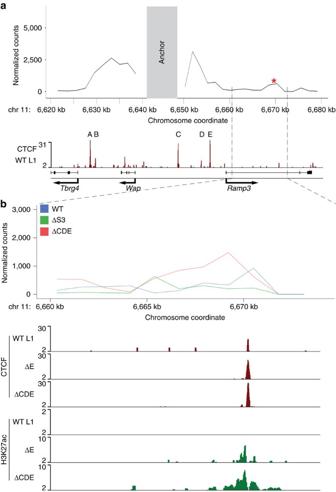Figure 6: Interactions between theWapsuper-enhancer and the first intron ofRamp3. (a) 4C data at theTbrg4-Wap-Ramp3locus were obtained from wild type lactating mammary tissue. The anchor region located over the third enhancer (S3) is shaded in grey. The lower panel shows CTCF-binding sites in theTbrg4-Wap-Ramp3locus. 4C interactions occurred between the first intron ofRamp3and the anchor region (red asterisk). (b) 4C signal within the first intron ofRamp3. Intronic 4C interactions in wild type (blue) were absent in ΔS3 mutants (green) and increased in ΔCDE mutants (red). The lower panel shows increased CTCF binding to the intronic site in ΔE and ΔCDE mutants along with an increase in H3K27ac. Full size image Figure 6: Interactions between the Wap super-enhancer and the first intron of Ramp3 . ( a ) 4C data at the Tbrg4 - Wap - Ramp3 locus were obtained from wild type lactating mammary tissue. The anchor region located over the third enhancer (S3) is shaded in grey. The lower panel shows CTCF-binding sites in the Tbrg4 - Wap - Ramp3 locus. 4C interactions occurred between the first intron of Ramp3 and the anchor region (red asterisk). ( b ) 4C signal within the first intron of Ramp3 . Intronic 4C interactions in wild type (blue) were absent in ΔS3 mutants (green) and increased in ΔCDE mutants (red). The lower panel shows increased CTCF binding to the intronic site in ΔE and ΔCDE mutants along with an increase in H3K27ac. Full size image RNAs associated with enhancers (eRNAs) tend to reflect their activities [43] . To determine whether increased expression of Ramp3 in mammary tissue lacking CTCF site E was caused by altered Wap super-enhancer activity, we examined eRNA levels. Total RNA-seq established the eRNA pattern over S3, the predominant constituent enhancer within the super-enhancer ( Fig. 7 ). Transcripts coincided with S3 and two additional STAT5-binding sites, which were also associated with H3K27ac marks as well as Pol II binding. Using 5′ and 3′ RACE we determined the exact structure of the eRNA emanating from S3 ( Fig. 7a , Supplementary Note 2 ). S3 eRNA levels were determined by qRT–PCR and no significant differences were observed between wild type and the three mutant tissues ( Fig. 7b ). This suggests that loss of CTCF sites flanking the super-enhancer does not affect its overall activity but rather extends its sphere of influence. 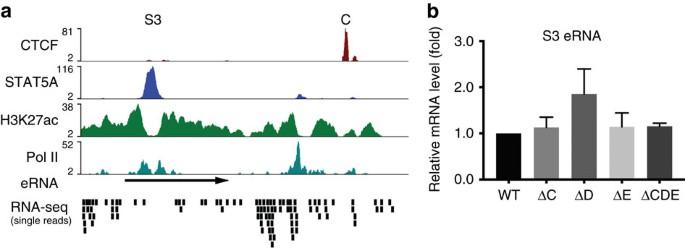Figure 7:Wapsuper-enhancer eRNA levels are independent of CTCF sites. (a) Structure of the S3 region of the super-enhancer. Site S3 is characterized by STAT5 binding, extensive H3K27ac, Pol II binding (GSE74826) and the presence of eRNAs (based on total RNA-seq data). Transcripts coincided with site S3 and additional STAT5-binding sites. An eRNA associated with S3 was identified and characterized using 5′ and 3′ RACE (Supplementary Note 2). (b) No statistically significant differences in S3 eRNA levels between mammary tissue from wild type and the mutants were observed. One-way ANOVA with multiple comparison and alpha 0.01 was applied (P=0.26). Results are shown as the means±s.e.m. of independent biological replicates; ΔCn=9 (−/−); ΔDn=5 (−/−); ΔEn=6 (−/−); ΔCDEn=3 (−/−). Figure 7: Wap super-enhancer eRNA levels are independent of CTCF sites. ( a ) Structure of the S3 region of the super-enhancer. Site S3 is characterized by STAT5 binding, extensive H3K27ac, Pol II binding (GSE74826) and the presence of eRNAs (based on total RNA-seq data). Transcripts coincided with site S3 and additional STAT5-binding sites. An eRNA associated with S3 was identified and characterized using 5′ and 3′ RACE ( Supplementary Note 2 ). ( b ) No statistically significant differences in S3 eRNA levels between mammary tissue from wild type and the mutants were observed. One-way ANOVA with multiple comparison and alpha 0.01 was applied ( P =0.26). Results are shown as the means±s.e.m. of independent biological replicates; ΔC n =9 (−/−); ΔD n =5 (−/−); ΔE n =6 (−/−); ΔCDE n =3 (−/−). Full size image Elevated Wap enhancer interactions upon loss of CTCF sites To understand the mechanism underlying the activation of Ramp3 in mammary tissue, especially upon loss of the three CTCF-binding sites separating it from the Wap super-enhancer, we conducted 4C experiments. Using the Wap super-enhancer as anchor we determined the interactions inherent to the native locus and elevated or de novo interactions obtained upon loss of CTCF sites ( Fig. 6 ). We investigated whether the Wap super-enhancer interacts with the Ramp3 gene and 4C experiments in wild type tissue demonstrated interactions of the S3 region with the Ramp3 gene ( Fig. 6a ). In accordance with our previous findings this interaction was abrogated in ΔS3 mutant mammary tissue. Upon deletion of all CTCF sites separating the Wap super-enhancer from Ramp3 , elevated interactions between the S3 region and the first intron of Ramp3 were detected ( Fig. 6b , upper panel). The underlying region coincided with augmented H3K27ac coverage ( Figs 5a and 6b , bottom panel) and increased CTCF binding in ΔCDE mutants ( Fig. 6b , centre panel). CTCF sites ensure Ramp3 expression in non-mammary tissues A characterizing feature of the Wap locus is its absolute silence in non-mammary tissues, which, however, soundly express the neighbouring Ramp3 . The presence of H3K4me3 marks on the Ramp3 promoter in non-mammary cells and tissues ( Fig. 8a ) provides evidence of its activity. This opened the possibility of the three CTCF sites shielding Ramp3 regulatory elements and thereby ensuring the silence of Wap in non-mammary cells. We initially addressed this question in the cerebellum, a tissue characterized by high Ramp3 expression and the absence of any detectable Wap mRNA. ChIP-seq analysis had demonstrated that from the three CTCF sites only site E was bound by CTCF in the cerebellum ( Fig. 2b ). Individual absence of CTCF sites D or E, nor the combined absence of sites C, D and E, failed to activate Wap ( Fig. 8b,c ). This demonstrates an inability of Ramp3 regulatory elements to spread into the Wap locus in non-mammary cells. Notably, deletion of CTCF site E resulted in a 90% reduction of Ramp3 mRNA levels in the cerebellum ( Fig. 8c ). The combined deletion of all three sites also led to a 90% reduction of Ramp3 . Similarly, reduced expression was also observed in other non-mammary tissues ( Fig. 8d ), including kidney and uterus. Finally, we investigated the possibility that CTCF site E coincides with putative regulatory elements. ChIP-seq data demonstrated the presence of strong DNase I hypersensitivity coinciding with CTCF site E and non-mammary cells ( Fig. 8e ). 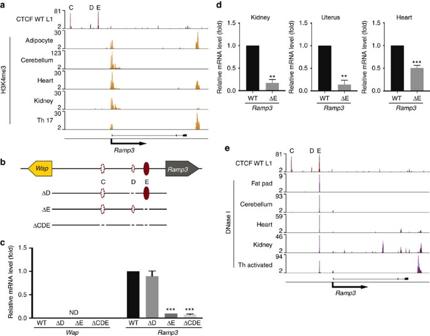Figure 8: Border CTCF site is required forRamp3expression in non-mammary cells. (a) H3K4me3 marks at theRamp3promoter indicated active transcription in several non-mammary cell types and tissues (GSE29218, GSE31039, GSE32864). (b) Out of the three CTCF-binding sites in mammary tissue that separate theWapsuper-enhancer andRamp3, only site E (filled crimson ovals) was present in non-mammary tissue, like cerebellum, heart, kidney and uterus. CTCF binding to sites C and D was absent in those tissues (dashed crimson ovals) (c) Deletion of site E as well as the combined deletion of sites C, D and E led to a 90% reduction inRamp3expression in the cerebellum. Deletion of site D did not affectRamp3expression. Results are shown as the means±s.e.m. of independent biological replicates; ΔD:n=3 (−/−); ΔE:n=6 (−/−); ΔCDE:n=4 (−/−); data were normalized toGapdh; one-way ANOVA with multiple comparison and alpha 0.01 was applied. *P<0.01, **P<0.001, ***P<0.0001. (d) Deletion of site E led to a significant reduction inRamp3expression in several non-mammary cells. Results are shown as the means±s.e.m. of independent biological replicates; Kidney and Uterus ΔE:n=3 (−/−); Heart ΔE:n=4 (−/−); data were normalized toGapdh; a two-tailed Student’st-test with alpha 0.01 was applied. *P<0.01, **P<0.001, ***P<0.0001. (e) CTCF site E coincided with DNase I hypersensitivity. Sites C and D were not occupied by CTCF in non-mammary cells and no DNase I hypersensitivity had been detected at these sites (GSE37074). Figure 8: Border CTCF site is required for Ramp3 expression in non-mammary cells. ( a ) H3K4me3 marks at the Ramp3 promoter indicated active transcription in several non-mammary cell types and tissues (GSE29218, GSE31039, GSE32864). ( b ) Out of the three CTCF-binding sites in mammary tissue that separate the Wap super-enhancer and Ramp3 , only site E (filled crimson ovals) was present in non-mammary tissue, like cerebellum, heart, kidney and uterus. CTCF binding to sites C and D was absent in those tissues (dashed crimson ovals) ( c ) Deletion of site E as well as the combined deletion of sites C, D and E led to a 90% reduction in Ramp3 expression in the cerebellum. Deletion of site D did not affect Ramp3 expression. Results are shown as the means±s.e.m. of independent biological replicates; ΔD: n =3 (−/−); ΔE: n =6 (−/−); ΔCDE: n =4 (−/−); data were normalized to Gapdh ; one-way ANOVA with multiple comparison and alpha 0.01 was applied. * P <0.01, ** P <0.001, *** P <0.0001. ( d ) Deletion of site E led to a significant reduction in Ramp3 expression in several non-mammary cells. Results are shown as the means±s.e.m. of independent biological replicates; Kidney and Uterus ΔE: n =3 (−/−); Heart ΔE: n =4 (−/−); data were normalized to Gapdh ; a two-tailed Student’s t -test with alpha 0.01 was applied. * P <0.01, ** P <0.001, *** P <0.0001. ( e ) CTCF site E coincided with DNase I hypersensitivity. Sites C and D were not occupied by CTCF in non-mammary cells and no DNase I hypersensitivity had been detected at these sites (GSE37074). Full size image In some cell types the presence of H3K27me3 marks has been linked to gene inactivity [44] , [45] and along with that, CTCF is known to separate active from repressive chromatin marks [7] , [46] , [47] . We therefore investigated the possibility that suppressive H3K27me3 marks in the Wap locus of non-mammary cells would spread into the active Ramp3 locus upon deletion of the CTCF sites. Based on ChIP-seq analyses [48] there were few, if any, H3K27me3 marks in the Wap-Ramp3 locus of mammary tissue ( Fig. 9a ). The Hoxα locus served as a positive control ( Fig. 9b ). Notably, in cerebella the Wap locus was also devoid of H3K27me3 marks ( Fig. 9c ), suggesting the inactivity of the Wap gene cannot be contributed to the presence of known suppressive marks. The Hoxα locus served as a positive control ( Fig. 9d ). Thus, silencing of Ramp3 in non-mammary tissues from mutant mice lacking the CTCF sites cannot be explained by the spreading of known silencing chromatin marks [47] , [49] , [50] , [51] , [52] . 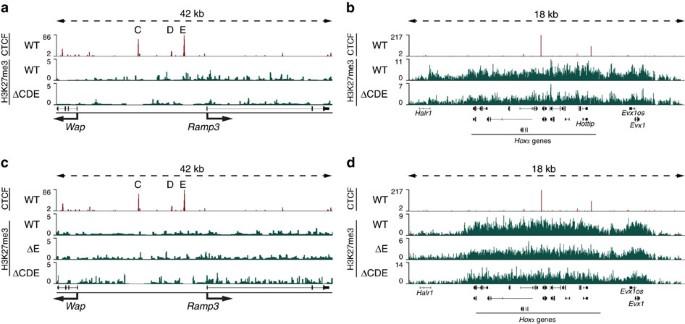Figure 9: Absence of K3K27me3 marks in theWap-Ramp3locus in mammary tissue and cerebellum. (a) H3K27me3 marks were virtually absent in theWap-Ramp3locus in mammary tissue from WT and ΔCDE mutants. (b) TheHoxαlocus served as a control locus and showed extensive H3K27me3 coverage in mammary tissue. (c) No increase of H3K27me3 marks in ΔE and ΔCDE mutants in the cerebellum. (d) TheHoxαlocus served as a control locus in the cerebellum and showed strong H3K27me3 coverage. Figure 9: Absence of K3K27me3 marks in the Wap-Ramp3 locus in mammary tissue and cerebellum. ( a ) H3K27me3 marks were virtually absent in the Wap - Ramp3 locus in mammary tissue from WT and ΔCDE mutants. ( b ) The Hoxα locus served as a control locus and showed extensive H3K27me3 coverage in mammary tissue. ( c ) No increase of H3K27me3 marks in ΔE and ΔCDE mutants in the cerebellum. ( d ) The Hoxα locus served as a control locus in the cerebellum and showed strong H3K27me3 coverage. Full size image Although a fundamental role of CTCF in shielding genetic neighbourhoods in ESCs had been established [7] , [18] , its ability to safeguard exceptionally strong cell-specific super-enhancers had not been investigated. Nor was it known whether CTCF enabled cell-specific genes to maintain a state of silence in non-target cells. Our findings emphasize more complex, and likely cell-specific, roles of CTCF sites and insulated neighbourhoods at the mammary-specific Wap locus that is activated by a cytokine-sensing super-enhancer during pregnancy [6] . Our in vivo study demonstrates, for the first time, that a cell-specific super-enhancer extends its functional reach beyond its respective target and past several CTCF sites into a juxtaposed neighbourhood where it activates a secondary target gene. Although these CTCF sites, including the loop anchor, do not block the super-enhancer, their deletion from the mouse genome demonstrates the capacity to muffle gene activation. We also demonstrate that these CTCF sites are essential for the expression of the neighbouring Ramp3 gene in non-mammary cells but are not required for the maintenance of transcriptional silence of Wap in non-mammary cells. Although deletion of CTCF sites separating enhancers from non-target genes can result in their activation, it appears that in ESCs [7] mainly those genes respond that are expressed at very low levels (FPKM/RPKM) [7] , [10] , [16] , [18] , [53] . In contrast, the mammary super-enhancer not only activates its native Wap gene but also bypasses several CTCF sites to further activate Ramp3 , a secondary target gene. This secondary target gene is located in a separate insulated neighbourhood and expressed across cell types. Thus, CTCF sites can muffle, but do not block, very strong enhancers. Moreover, loss of CTCF sites permits mammary enhancers to only induce genes that already display some baseline activity but not silent genes [30] . Although the activation of genes upon loss of CTCF sites is generally attributed to de novo promoter–enhancers interactions [16] , [28] , [30] , [54] , [55] , [56] , the mammary enhancer in this study establishes interactions with a dormant CTCF-binding site within the first intron of the neighbouring genes, which leads to the deposition of activating H3K27ac marks. While it is not clear why CTCF sites and loop anchors vary in their insulating strength [57] , the presence of several CTCF sites might increase the “insulation score” [8] . Two hundred and seventy out of the 440 mammary-specific super-enhancers have more than one CTCF site as a boundary to the neighbouring genes, which would increase their insulation score. The ability of enhancers to activate genes over great distances and independent of their location with respect to promoters is a core dogma [58] that is largely based on studies conducted outside the native genomic environment. However, in vivo rules guiding enhancers to pair up with their respective target genes are more complex [58] and the ‘search space’ of enhancers might be confined to TADs and insulated neighbourhoods [59] , [60] . Notably, while the Wap super-enhancer activates its own gene and the juxtaposed Ramp3 located in a separate neighbourhood, it has little or no capacity to reach over its own target and activate the downstream Tbrg4 gene even upon deletion of the two separating CTCF sites. This suggests that the search space of enhancers might not extend past its nearest promoters [61] , [62] , [63] . Boundaries that establish insulated neighbourhoods are required to maintain repression of specific gene sets in ESCs [7] and deletion of anchor CTCF sites leads to their inappropriate activation [7] . Although this mechanism is operative in Polycomb-repressed genes in ESCs, it does not apply to the mammary-specific Wap gene and possibly not to other genes controlled by mammary super-enhancers. While genes regulated by mammary-specific enhancers are silent in non-mammary cells, they do not display visible repressive H3K27me3 marks in non-expressing cells [48] . Loss of the CTCF neighbourhood anchor at the widely expressed Ramp3 gene fails to awaken the juxtaposed silent Wap gene in non-mammary cell types, but it rather leads to the suppression of Ramp3 expression. Thus, CTCF sites bordering the mammary super-enhancer serve two distinct functions, limiting its exposure to the neighbouring Ramp3 gene in mammary epithelium and permitting Ramp3 expression in non-mammary cells. At this point it is not clear whether CTCF boundaries associated with other cell-specific super-enhancers also exhibit such dual functions. In summary, our study suggests more complex and cell-specific functions of CTCF sites associated with exceptionally strong lineage-restricted super-enhancers. Generation of mutant mice CRISPR/Cas9 targeted mice were generated by the transgenic core of the National Heart, Lung, and Blood Institute (NHLBI). Single-guide RNAs (sgRNA) were designed using MIT’s CRISPR Design tool ( http://crispr.mit.edu/ ). Those spanning CTCF-binding sites were synthesized (OriGene, Thermo Fisher Scientific). The sgRNAs were injected with Cas9 protein into the cytoplasm of fertilized eggs from C57BL/6 × C57BL/6 mating and transplanted into pseudopregnant C57BL/6 mice to obtain founders. Sequences of the sgRNA used can be found in Supplementary Table 1 . Mice carrying loxP sites flanking CTCF sites A and B were generated by InGenious using homologous recombination. The sequences between loxP sites were deleted using the germline Figla-Cre delete mice (gift from Jurrien Dean, NIDDK, NIH). Genotyping and generation of homozygous mutant mice All animal procedures were in accordance with NIH, NIDDK guidelines for the care and use of laboratory animals. Founders, many of them mosaic, were bred with C57BL/6 wild type mice to segregate the various mutant alleles. Tail snips were taken from mice and genotyped by genomic DNA PCR. The PCR products were analysed by Sanger sequencing. Primer information can be found in Supplementary Table 2 . Once mutant alleles were identified and characterized, F1 mice were inbred to obtain homozygous mice. The mouse lines generated by CRISPR/CAS9 gene editing and used in this study carried the following deletions: line ΔC (58 bp), ΔD (134 bp), ΔE (160 bp) and ΔCDE (ΔC 2,442 bp; ΔD 4 bp; ΔE 1,165 bp). The deletion of line ΔAB is 1,711 bp. The specific deletion of each line can be found in the Supplementary Note 1 . RNA isolation and qRT–PCR Total RNA was isolated using the PureLink RNA Mini kit (Ambion) per the manufacturer’s protocol and cDNA was synthesized from 1 μg RNA using oligo dT primers and SuperScript II/III (Invitrogen). Quantitative TaqMan PCR was performed in triplets on the CFX384 Real-Time PCR Detection System (Bio-Rad) using the following probes: Tbrg4 Mm01220234_g1; Wap Mm00839913_m1; Ramp3 Mm00840142_m1; Gapdh 4352339E of Applied Biosystems. Ct-values were normalized to the housekeeping gene Gapdh and fold-changes were calculated using the comparative Ct-method (2 −ΔΔCt method). RACE RACE assay was done using the FirstChoice RLM-RACE Kit (Ambion) according to the manufacturer’s instructions. The following primers were used in the nested PCRs in the assay. 5′RACE, Outer Primer 5′-CTCTTCCACCCTGTCCACTGCTC-3′; Inner Primer 5′-AGAGTTGATGGGGCAGGAAAGAGCC-3′. 3′RACE, Outer Primer 5′-CACATAGTAGCCGAGGATGGCC-3′; Inner Primer 5′-GGCACCTGCCTCCTCCTTCTAGTCT-3′. The PCR products were then purified and sequenced to identify the 5′ and 3′ end of eRNA transcript ( Supplementary Note 2 ). ChIP-seq Mammary tissues were collected on day one of lactation (L1) and cerebella from 2- to 11-month-old female mice. For cerebellum ChIP, four cerebella were pooled per biological replicate. All tissues were snap frozen and stored at −80 °C. Tissues were pulverized in liquid nitrogen followed by chromatin fixation with 1% formaldehyde final concentration. Washed chromatin (PBS) was homogenized using a dounce tissue grinder in Farnham’s lysis buffer and followed by chromatin fragmentation through sonication. Fragmentation efficiency in the range of 200–500 bp was controlled by gel electrophoresis and ChIP was performed using 50 μl Dynabeads Protein A (Invitrogen) and 10 μg of the following antibodies per ChIP (Manufacturer, Catalogue Number): anti-CTCF (Abcam, ab70303), anti-H3K27ac (Abcam, ab4729), anti-H3K27me3 (Abcam, ab6002). Ten microlitres of anti-CTCF (Millipore, 07-729) was used (no concentration provided by Millipore). Indexed libraries were produced using the NEBNext Ultra II DNA Library Prep Kit and NEBNext Index Primer Set for Illumina according to the manufacturer’s protocol. Fragments between 200 and 500 bp were selected by gel electrophoresis and 50 bp single-end sequencing was performed on an Illumina HiSeq 2500. Total RNA-seq Total RNAs were extracted from mammary tissue at day 18 of pregnancy and purified twice with Trizol and RNeasy Plus Mini Kit (Qiagen, 74134). Ribosomal RNA was removed from 1 μg of total RNAs and cDNA was synthesized using SuperScript II (Invitrogen). Libraries for sequencing were prepared according to the manufacturer’s instructions with TruSeq Stranded Total RNA Library Prep Kit with Ribo-Zero (Illumina, RS-122-2201) and paired-end sequencing was done with a HiSeq 2000 instrument (Illumina). Circular chromosome conformation capture (4C)-seq The 4C protocol was adapted from published methods [64] , [65] . Frozen-stored mammary tissues collected at L1 were ground into powder. Chromatin was fixed with formaldehyde (final 1%) for 15 min at room temperature, and then was quenched with glycine (final 0.125 M). Pellets were lysed in lysis buffer (10 mM Tris HCI pH 8.0, 10 mM NaCl, 0.5% Nonidet P-40) containing phenylmethylsulfonyl fluoride and protease inhibitors, incubated on ice for 30 min, and dounced using a pre-chilled glass homogenizer, followed by another 10 min incubation on ice. After removal of supernatant, nuclei pellets were re-suspended in DpnII buffer (New England Biolabs). SDS was added to a final concentration of 0.2% and samples were incubated for 1 h at 37 °C. Two per cent Triton X-100 was added, followed by incubation for 1 h at 37 °C. Samples were incubated with 400 units each of restriction enzymes DpnII (New England Biolabs) and were incubated overnight at 37 °C. To enzyme inactivation SDS was added (final 1%) and incubated for 30 min at 65 °C, followed by SDS-sequestration with 1% Triton X-100 at 37 °C for 1 h, T4 ligase (New England Biolabs) was added to each sample and incubated for overnight at 16 °C. Ligated samples were treated overnight with proteinase K (20 mg ml −1 , Invitrogen) at 65 °C and 1 h at 37 °C with RNase A (10 mg ml −1 , Thermo Fisher Scientific), and DNA fragments were purified by phenol–chloroform method. DNA fragments from 3C were digested with Mse I (New England Biolabs) overnight at 37 °C and ligated using T4 ligase overnight at 16 °C. DNA was purified by phenol/chloroform method and then amplified with site-specific primers linked to the Illumina DNA adaptors. Libraries for next generation sequencing were prepared and sequenced with HiSeq 2500 (Illumina). ChIP-seq analysis ChIP-seq data were analysed using Trimmomatic [66] (version 0.33), for quality check and removal of low-quality reads (parameters: LEADING: 20, TRAILING: 20, SLIDINGWINDOW: 4:20, MINLEN: 20, HEADCROP: 15), and Bowtie aligner [67] (version 1.1.2) with the −m 1 parameter to obtain only uniquely mapped reads, except for CTCF samples where the −m 3 and best parameters were used. Reads were mapped to the reference genome mm10. For ChIP-seq data from GEO, Trimmomatic [66] (version 0.33) was used to check read quality (using the following parameters: LEADING: 3, TRAILING: 3, SLIDINGWINDOW: 4:20, MINLEN: 20). The alignment was performed applying Bowtie aligner [67] (version 1.1.2) using −m 1 as the parameter. HOMER software [68] (default settings) and Integrative Genomics Viewer [69] (IGV) were applied for visualization. MACS2 (ref. 70 ) peak finding algorithm (version 2.1.0) was used to identify regions of ChIP-seq enrichment over background. For further analyses additional tools were used [68] , [71] , [72] . DNase-seq analysis DNase-seq data were treated as described [73] . The reads were trimmed to the first 20 bp using Trimmomatic [66] and bwa [74] (default setting) was used for alignment to mm10. Further visualization was done with Homer [68] and IGV [69] . mRNA-seq analysis RNA-seq data were trimmed using Trimmomatic [66] (parameters: LEADING: 20, TRAILING: 20, SLIDINGWINDOW: 4:20, MINLEN: 20, HEADCROP: 15) and mapped using a STAR RNA-seq aligner [75] (default settings, GRCm38.84 as a GTF file). The GTF file was filtered, by excluding predicted genes (LOC, Rik and BC), to retain only high-confident genes. RNA-seq analyses were done using R (version 3.2.3), Bioconductor [76] , and the packages Rsubread [77] and DESeq2 (ref. 78 ). Total RNA-seq analysis Total RNA-seq reads were analysed using Trimmomatic [66] (version 0.33) to check read quality (with following parameters: LEADING: 3, TRAILING: 3, SLIDINGWINDOW: 4:20, MINLEN: 36). The alignment was performed in the Bowtie aligner [67] (version 1.1.2) using paired end mode. 4C-seq data analysis The sequencing data were processed using the 4C-ker [79] . All 4C-seq images were generated using 4Cker R package with k =4 and k =6. Statistical analyses The samples for qRT–PCR and ChIP-seq were randomly, but not blinded, selected. Statistical analysis of qRT–PCR and RNA-seq data was performed as follows. Data were analysed for normal distribution using Shapiro–Wilk normality test and statistical power was calculated with a significance level of 0.01 and a statistical power of 0.9. Power calculations were adapted for two-sample t -tests and one-way ANOVA analyses. Statistical significance between two groups was calculated using a two-tailed Student’s t -test with a confidence level of 99%. For comparison between more than two groups, one-way ANOVA was used with a confidence level of 99%. Analyses were done in R and GraphPad Prism (version 7.0a). URLs MIT CRISPR Design tool, http://crispr.mit.edu/; R Project for Statistical Computing, https://www.R-project.org/ and dplyr ( https://CRAN.R-project.org/package=dplyr ). Data availability ChIP-seq, RNA-seq and 4C-seq data are available at NCBI’s Gene Expression Omnibus (GEO). The SuperSeries is accessible under GSE92932, comprising ChIP-seq under the accession number GSE92587, RNA-seq under GSE92931 and 4C-seq under GSE97803. Already published ChIP-seq, DNase-seq and RNA-seq data were taken from GEO: GSE29218, GSE31039, GSE32864, GSE37074, GSE37646, GSE40918, GSE74189, GSE74826, GSE92590, GSE90788. Hi-C and ChIA-PET data are available under GSE35156 and GSE57911, respectively. How to cite this article: Willi, M. et al . Facultative CTCF sites moderate mammary super-enhancer activity and regulate juxtaposed gene in non-mammary cells. Nat. Commun. 8 , 16069 doi: 10.1038/ncomms16069 (2017). Publisher’s note: Springer Nature remains neutral with regard to jurisdictional claims in published maps and institutional affiliations.